miR-195/497 induce postnatal quiescence of skeletal muscle stem cells Skeletal muscle stem cells (MuSCs), the major source for skeletal muscle regeneration in vertebrates, are in a state of cell cycle arrest in adult skeletal muscles. Prior evidence suggests that embryonic muscle progenitors proliferate and differentiate to form myofibres and also self-renew, implying that MuSCs, derived from these cells, acquire quiescence later during development. Depletion of Dicer in adult MuSCs promoted their exit from quiescence, suggesting microRNAs are involved in the maintenance of quiescence. Here we identified miR-195 and miR-497 that induce cell cycle arrest by targeting cell cycle genes, Cdc25 and Ccnd . Reduced expression of MyoD in juvenile MuSCs, as a result of overexpressed miR-195/497 or attenuated Cdc25/Ccnd, revealed an intimate link between quiescence and suppression of myogenesis in MuSCs. Transplantation of cultured MuSCs treated with miR-195/497 contributed more efficiently to regenerating muscles of dystrophin-deficient mice, indicating the potential utility of miR-195/497 for stem cell therapies. The regenerative capacity of adult skeletal muscle is attributed to skeletal muscle stem cells (MuSCs), which are called satellite cells because of their location underneath the basal lamina of muscle fibres. Adult MuSCs are normally quiescent, in cell cycle arrest, and they only re-enter the cell cycle on muscle damage, either by injury or under pathological conditions such as Duchenne muscular dystrophy (DMD). They then proliferate and enter the regenerative myogenic programme, giving rise to differentiated skeletal muscle cells forming myofibres, and also generating a renewed population of quiescent MuSCs. In this study, we asked how adult MuSCs establish and maintain their quiescent state. Previous studies revealed the involvement of key transcription factors in the establishment of MuSCs. Embryonic myogenic progenitor cells that express the paired box transcription factors, Pax3 and its paralogue Pax7, enter the skeletal muscle programme when they begin to express the myogenic determination factors, Myf5 and MyoD [1] . This population of Pax3/7-positive progenitors is essential for skeletal muscle growth during development and also considered to be the source of adult MuSCs [2] , [3] , [4] , [5] . The expression of Pax7 is essential for the establishment and maintenance of adult MuSCs [6] , [7] , [8] . Most of these MuSCs are primed for myogenesis by the activation of myogenic regulatory factors during development [9] , [10] , [11] . While genetic evidence suggests that adult MuSCs have previously activated the MyoD gene and are thus primed for myogenesis, the MyoD protein is not detectable in quiescent MuSCs, until they are activated for regenerative myogenesis on injury [12] , [13] . Thus, Pax3/Pax7-positive proliferating progenitor cells have entered the myogenic programme, and become Pax7-positive/MyoD protein-negative (Pax7+/MyoD protein-) quiescent MuSCs in adult skeletal muscle [14] . We found that the juvenile to adult transition is accompanied by the downregulation of MyoD protein in MuSCs. The comparison between MuSCs isolated from juvenile and adult mice led us to identify microRNAs (miRNAs) that convert proliferating juvenile MuSCs into a cell cycle arrested state through targeting genes for cell cycle progression. The absence of MyoD protein in these Pax3/7-positive cells suggests a close link between quiescence and suppression of myogenesis in adult MuSCs. Manipulation of the activity of these miRNAs shows that they can improve the regenerative efficiency of cultured MuSCs on transplantation into pathological muscle. Adult MuSCs acquire quiescence later during development We first determined the periods when myogenic priming occurs for the MyoD gene in green fluorescent protein (GFP)-positive (GFP+) cells isolated from Pax3 GFP/+ ; MyoD-Cre; Rosa26 CAG-LSL-RFP/+ compound mice [15] ( Supplementary Fig. 1 ). These GFP+, Pax3-expressing MuSCs isolated from adult skeletal muscle have sustained expression of red fluorescent protein (RFP) once the MyoD gene has been activated in these mice. By separating Pax3GFP; MyoD-primed RFP double-positive (GFP+RFP+) from only GFP+ (GFP+RFP−) cells by flow cytometry, from embryonic day 16.5 to 6 months old adult mice, we confirmed that almost all GFP+ MuSCs in the diaphragm muscle, where Pax3GFP is highly expressed than in limb muscle during perinatal stages [12] , were primed for the MyoD gene by 12 weeks ( Fig. 1a and Supplementary Fig. 1d ). In contrast, about half of prenatal and neonatal GFP+ cells have not been primed for myogenesis as indicated by the lack of activation of the MyoD gene in diaphragm muscles ( Fig. 1a ). When these embryonic and neonatal GFP+RFP− (not MyoD primed) cells were cultured ex vivo , GFP intensity gradually decreases, accompanied by the activation of MyoD-primed RFP, showing that these embryonic and neonatal GFP+RFP− cells are still in a pre- MyoD -primed state ( Supplementary Fig. 1e–g ). Analysis by fluorescence-activated cell sorting showed that the ratio of RFP+ cells in the population of GFP+ cells increased gradually in juvenile mice (1–3 weeks) before reaching a plateau at 12 weeks. The majority of freshly isolated GFP+RFP+ cells still translates MyoD protein in juvenile mice, while MyoD protein is not detected in freshly isolated GFP+RFP+ cells from adult mice ( Fig. 1b–e and Supplementary Fig. 1h,i ), suggesting that GFP+ cells are primed for MyoD gene transcription at juvenile stages before downregulating MyoD protein during the juvenile to adult phase transition. 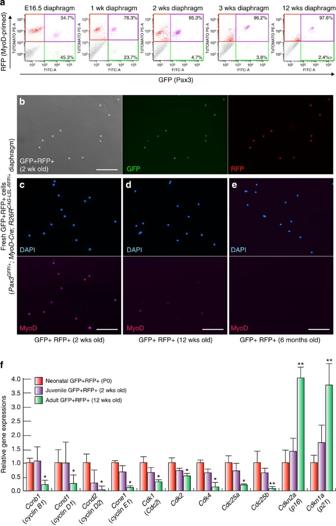Figure 1: Alteration of gene expression in MuSCs during the juvenile to adult transition. (a) Representative fluorescence-activated cell sorting profiles with Pax3-GFP and MyoD-primed RFP double-positive (GFP+RFP+, purple) cells of diaphragms from embryonic day (E) 16.5–12 weeks (wks) old mice. (b–e) The expression of MyoD protein in GFP+RFP+ MuSCs during the juvenile to adult transition. Freshly isolated GFP+RFP+ cells at different ages were evaluated by immunofluorescent staining with antibody against MyoD (labelled with Alexa647, pink). GFP+RFP+ cells from 2-week-old mice (b) express MyoD protein (c), its expression is decreased in cells freshly isolated from 12 weeks (d) and 6 months old mice (e). Nuclei were stained with 4′,6-diamidino-2-phenylindole (DAPI) (blue inc–e). Scale bar, 50 μm. (f) The juvenile to adult transition is accompanied by a decrease in transcripts for cell cycle progression genes and the increase in those for cell cycle arrest in GFP+RFP+ cells from the diaphragm muscle. Representative RT–qPCR of cell cycle transcripts is shown. All error bars indicate ±s.e.m. (n=3).Pvalues are determined byt-test from a two-tailed distribution. *P<0.05; **P<0.01. Figure 1: Alteration of gene expression in MuSCs during the juvenile to adult transition. ( a ) Representative fluorescence-activated cell sorting profiles with Pax3-GFP and MyoD-primed RFP double-positive (GFP+RFP+, purple) cells of diaphragms from embryonic day (E) 16.5–12 weeks (wks) old mice. ( b – e ) The expression of MyoD protein in GFP+RFP+ MuSCs during the juvenile to adult transition. Freshly isolated GFP+RFP+ cells at different ages were evaluated by immunofluorescent staining with antibody against MyoD (labelled with Alexa647, pink). GFP+RFP+ cells from 2-week-old mice ( b ) express MyoD protein ( c ), its expression is decreased in cells freshly isolated from 12 weeks ( d ) and 6 months old mice ( e ). Nuclei were stained with 4′,6-diamidino-2-phenylindole (DAPI) (blue in c – e ). Scale bar, 50 μm. ( f ) The juvenile to adult transition is accompanied by a decrease in transcripts for cell cycle progression genes and the increase in those for cell cycle arrest in GFP+RFP+ cells from the diaphragm muscle. Representative RT–qPCR of cell cycle transcripts is shown. All error bars indicate ±s.e.m. ( n =3). P values are determined by t -test from a two-tailed distribution. * P <0.05; ** P <0.01. Full size image The absence of MyoD protein is one of the hallmarks of quiescent adult MuSCs [14] , [16] , [17] . Therefore, we next examined whether the juvenile to adult phase transition is accompanied by a change in GFP+RFP+ cells from an actively proliferating to a non-proliferating quiescent state. GFP+RFP+ cells freshly isolated from juvenile mice (2 weeks old) included a much higher ratio of Ki67+ cells than in adult (12 weeks old) MuSCs ( Fig. 2b,c ). Moreover, large differences in gene expression for some regulators of the cell cycle were observed between GFP+RFP+ cells freshly isolated from juvenile and those from adult mice, however, not between those from neonatal (P0) and juvenile mice. The expression of genes for cell cycle activators, including cyclin families ( Ccnb1, Ccnd1, Ccnd2, Ccne1 ), cyclin-dependent kinases ( Cdk1, Cdk2, Cdk4 ) and cell cycle division families ( Cdc25a, Cdc25b ) was strongly decreased. Conversely, expression of genes for cyclin-dependent kinase inhibitors Cdkn2a (p16) and Cdkn1a (p21) was increased in adult GFP+RFP+ ( Fig. 1f ). Thus the quiescent state of MuSCs is regulated by mechanisms that are predominant in adult but not juvenile skeletal muscle. 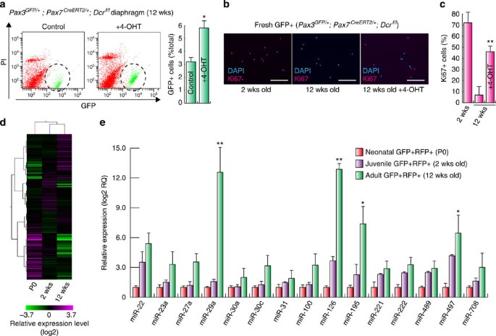Figure 2: Identification of upregulated miRNAs in adult MuSCs. (a–d) Aberrant proliferation of Dicer-inactivated adult MuSCs. (a) The fluorescence-activated cell sorting profiles of GFP+ cells with (left) and without (right panel) Dicer, isolated from the diaphragm of 12 weeks oldPax3GFP/+;Pax7CreER/+;Dcrf/fmice are shown. The proportion of GFP+ cells is increased in conditional Dicer-inactivated adult MuSCs. (b,c) GFP+ cells isolated from the diaphragm of 2-week-old mice are highly proliferating (Ki67-positive red cells inb), while those from the adult diaphragm are in a quiescent state. Conditional Dicer inactivation in adult MuSCs have spontaneously exited quiescence and entered the cell cycle. Nuclei were stained with 4′,6-diamidino-2-phenylindole (DAPI) (blue). Scale bar, 50 μm. (d) Heatmap of miRNA microarray data illustrating differentially expressed miRNA genes between GFP+RFP+ MuSCs in neonatal (P0), juvenile (2 weeks) and adult (12 weeks) mice. (e) miRNAs that increase strongly with age in GFP+RFP+ MuSCs. Representative RT–qPCR of miRNA transcripts in GFP+RFP+ MuSCs from neonatal (red), juvenile (purple) and adult (green) mice, normalized toRnu6. All error bars indicate ±s.e.m. (n=3).Pvalues are determined byt-test from a two-tailed distribution. *P<0.05; **P<0.01. Figure 2: Identification of upregulated miRNAs in adult MuSCs. ( a – d ) Aberrant proliferation of Dicer-inactivated adult MuSCs. ( a ) The fluorescence-activated cell sorting profiles of GFP+ cells with (left) and without (right panel) Dicer, isolated from the diaphragm of 12 weeks old Pax3 GFP/+ ; Pax7 CreER/+ ; Dcr f/f mice are shown. The proportion of GFP+ cells is increased in conditional Dicer-inactivated adult MuSCs. ( b , c ) GFP+ cells isolated from the diaphragm of 2-week-old mice are highly proliferating (Ki67-positive red cells in b ), while those from the adult diaphragm are in a quiescent state. Conditional Dicer inactivation in adult MuSCs have spontaneously exited quiescence and entered the cell cycle. Nuclei were stained with 4′,6-diamidino-2-phenylindole (DAPI) (blue). Scale bar, 50 μm. ( d ) Heatmap of miRNA microarray data illustrating differentially expressed miRNA genes between GFP+RFP+ MuSCs in neonatal (P0), juvenile (2 weeks) and adult (12 weeks) mice. ( e ) miRNAs that increase strongly with age in GFP+RFP+ MuSCs. Representative RT–qPCR of miRNA transcripts in GFP+RFP+ MuSCs from neonatal (red), juvenile (purple) and adult (green) mice, normalized to Rnu6 . All error bars indicate ±s.e.m. ( n =3). P values are determined by t -test from a two-tailed distribution. * P <0.05; ** P <0.01. Full size image miR-195/497 increase in adult MuSCs to induce cell cycle arrest We next asked whether miRNAs participate in the quiescence of adult MuSCs. There is evidence that non-coding RNAs, including miRNAs, are involved in the regulation of skeletal muscle cells during development [18] , [19] , [20] , [21] , [22] and of quiescent of MuSCs in the adult [10] , [22] , [23] , [24] . To examine the impact of miRNAs on the growth and differentiation of MuSCs, Dicer was deleted in Pax3/Pax7-expressing adult GFP+ cells of 12 weeks old Pax3 GFP/+ ; Pax7 CreER/+ ; Dcr f/f mice produced from Pax7 CreER/+ ; Dcr f/f female mice crossed with Pax3 GFP/+ ; Dcr f/f male mice, which did not reveal a haploinsufficient phenotype, by administration of 4-hydroxytamoxifen five times for a week ( Supplementary Fig. 2a–c ). Fluorescence-activated cell sorting analyses revealed that the number of GFP+ cells increased in Dicer -mutated diaphragms ( Fig. 2a ), and then decreased gradually, probably due to apoptosis [23] ( Supplementary Fig. 2d ). The percentage of Ki67+ cells in the population of GFP+ cells isolated from the diaphragm of adult mice was much lower than that in GFP+ cells of juvenile control mice. In contrast, GFP+ cells isolated from the diaphragm of adult mice after the conditional deletion of Dicer had a significantly higher percentage of Ki67+ cells than in the control adult GFP+ cells ( Fig. 2b,c ), suggesting the involvement of miRNAs in the suppression of cell proliferation in MuSCs. These results led us to explore miRNAs that cause the cell cycle arrest of MuSCs during the juvenile to adult phase transition. We performed miRNA microarray analyses with GFP+RFP+ cells isolated from diaphragms of neonatal, juvenile and adult mice. Reverse transcriptase quantitative PCR (RT–qPCR) analyses were performed to confirm the results. ( Fig. 2d,e , and Supplementary Table 1 ). Among miRNAs expressed in these cells, the expression level of miR-29a, miR-126, miR-195 and miR-497 was increased significantly with age in both miRNA microarray and RT–qPCR analyses. miR-31 (ref. 10 ), miR-489 (ref. 23 ) and miR-708 (ref. 25 ) were highly expressed in adult GFP+RFP+ cells. To determine whether any of the miRNAs upregulated in adult MuSCs controlled quiescence, individual miRNAs were transfected into GFP+RFP+ cells isolated from juvenile diaphragms of 2 weeks old mice and cultured for 3 days ( Supplementary Fig. 3a,b ). miR-29a and miR-126 did not significantly affect total numbers of cultured cells in each colony. In contrast, miR-195 and miR-497, members of the miR-15 family with the same seed sequence, strikingly inhibited the proliferation of cells, compared with control miRNA, after 3 days culture ( Supplementary Fig. 3b,c ). The introduction of either miR-195 or miR-497 led to a significant decrease in the incorporation of EdU ( Fig. 3a–d ) and in the ratio of phosphohistone H3 (pHH3)-positive cells of growing juvenile GFP+RFP+ cells ( Supplementary Fig. 4a,b ). The cell cycle profile analyses revealed that juvenile GFP+RFP+ cells accumulated in the G1(G0) and G2 phases after the introduction of miR-195 or miR-497, or both miR-195/miR-497 ( Supplementary Fig. 4c ), indicating that these miRNAs blocked the G1/S and G2/M transition of these cells preventing their progression into mitosis. As mentioned above, the quiescence of MuSCs during the juvenile to adult phase transition is accompanied by the reduction of MyoD protein ( Fig. 1c–e ). When either miR-195 or miR-497 were overexpressed in juvenile GFP+RFP+ cells, the ratio of MyoD protein+ cells was significantly lower than in cells overexpressing a control miRNA ( Fig. 3e–h ). Moreover, these cultured cells treated with miR-195/497, but not with control miRNA, showed a striking increase in the ratio of Pax7+MyoD− cells ( Fig. 3i–k ). miR-195/497 treatment caused a decrease of Ki67+ proliferating cells in both Pax7+ and MyoD+ cells. While the majority of Pax7+MyoD− cells are in a quiescent condition, MyoD+ cells remain proliferating, suggesting that the transition from proliferating to quiescent states of GFP+RFP+ MuSCs by miR-195/497 treatment leads to the increase in Pax7+ quiescent MuSC population ( Fig. 3l ). Thus, the quiescence induced in proliferating juvenile MuSCs with miR-195/497 was accompanied by an increase in the number of Pax7+MyoD− cells, characteristic of quiescent adult MuSCs. 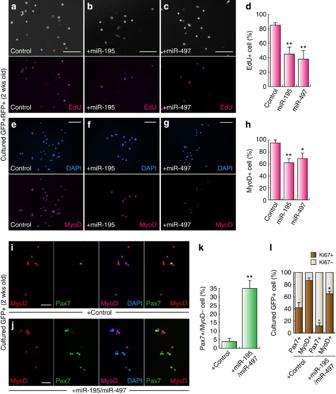Figure 3: miR-195 and miR-497 induce cell cycle exit in MuSCs. (a–d) Introduction of miR-195 or miR-497 causes cell cycle withdrawal in juvenile GFP+RFP+ cells cultured for 3 days. Cell cycle progression was evaluated by incorporation of EdU (labelled with Alexa647, pink). Scale bar, 50 μm. (e–k) miR-195 and miR-497 reduce the level of MyoD protein (labelled with Alexa647, pink ine–g,i,j, converted into red ini,j) and prevent downregulation of Pax7 (labelled with Alexa594, converted into green ini,j) in cultured GFP+(RFP+) cells isolated from 2-week-oldPax3GFP/+mice. Nuclei were stained with 4′,6-diamidino-2-phenylindole (DAPI) (blue). Scale bar, 50 μm (e–g) and 20 μm (i,j). (l) miR-195/497 attenuate proliferation in both Pax7+ and MyoD+ populations of cultured GFP+ cells isolated from 2-week-oldPax3GFP/+mice. All error bars indicate ±s.e.m. (n=3).Pvalues are determined byt-test from a two-tailed distribution. *P<0.05; **P<0.01. Figure 3: miR-195 and miR-497 induce cell cycle exit in MuSCs. ( a – d ) Introduction of miR-195 or miR-497 causes cell cycle withdrawal in juvenile GFP+RFP+ cells cultured for 3 days. Cell cycle progression was evaluated by incorporation of EdU (labelled with Alexa647, pink). Scale bar, 50 μm. ( e – k ) miR-195 and miR-497 reduce the level of MyoD protein (labelled with Alexa647, pink in e – g , i , j , converted into red in i , j ) and prevent downregulation of Pax7 (labelled with Alexa594, converted into green in i , j ) in cultured GFP+(RFP+) cells isolated from 2-week-old Pax3 GFP/+ mice. Nuclei were stained with 4′,6-diamidino-2-phenylindole (DAPI) (blue). Scale bar, 50 μm ( e – g ) and 20 μm ( i , j ). ( l ) miR-195/497 attenuate proliferation in both Pax7+ and MyoD+ populations of cultured GFP+ cells isolated from 2-week-old Pax3 GFP/+ mice. All error bars indicate ±s.e.m. ( n =3). P values are determined by t -test from a two-tailed distribution. * P <0.05; ** P <0.01. Full size image miR-195/497 target Cdc25 and Ccnd to maintain the stemness Two target prediction algorithms (TargetScan; www.targetscan.org/ and miRanda; www.microrna.org/ ) predicted 3′ untranslated regions (3′UTRs) of transcripts for the cell cycle genes Cdc25 and Ccnd as targets for the miR-15 family ( Supplementary Fig. 5,6 , Supplementary Data 1 and Supplementary Table 3 ). This led us to examine whether miR-195 and miR-497 regulate the messenger RNAs for these genes in MuSCs. Overexpression of miR-195 and miR-497 in GFP+RFP+ cells isolated from juvenile mice resulted in a significant decrease in transcript levels for Cdc25a, Cdc25b1/2 and Ccnd2 ( Fig. 4a ). To confirm whether miR-195/497 indeed affect messenger RNAs of these genes through interacting with putative target sites in the 3′UTR, intact and mutated 3′UTRs of these RNAs were cloned into luciferase reporters, and the constructs were co-transfected with or without pre-miR-195/497 expression constructs into HEK293T cells ( Supplementary Fig. 7 ). miR-195/497 down-regulated luciferase activities in the presence of wild-type, but not mutated, 3′UTRs of Cdc25a and Cdc25b messenger RNAs ( Fig. 4b ). Both 3′UTRs of Ccnd1 and Ccnd2 RNAs had two and three putative target sites respectively; site 3 of the Ccnd2 3′UTR was significantly targeted by miR-195/497 ( Fig. 4b and Supplementary Fig. 8 ). 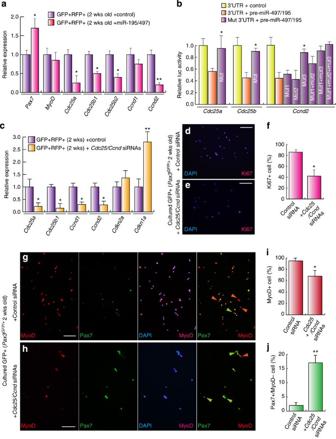Figure 4: miR-195/497 targetCdc25andCcndmessenger RNAs to induce the quiescence of MuSCs. (a) Effects of miR-195/497 administration on expression of genes for myogenic and cell cycle regulators in GFP+RFP+ cells isolated from diaphragms of 2-week-old mice. (b) Relative luciferase activity in 293T cells transfected with constructs of luciferase cDNA ligated to the 3′UTR or mutated 3′UTR (mut inCdc25a/b, mut1~3 inCcnd2) ofCdc25a,Cdc25bandCcnd2messenger RNAs, with or without pre-miR-497/195. (c–f) Introduction of mixed siRNAs againstCdc25andCcndcauses cell cycle exit in juvenile GFP+(RFP+) MuSCs. (c) Relative transcription levels of cell cycle regulators in cultured GFP+RFP+ cells of 2-week-old mice treated with or without the mixture ofCdc25andCcndsiRNAs are shown, indicating effective suppression of cell cycle progression with these siRNAs. (d–f) Effects of siRNAs againstCdc25andCcndtranscripts on the ratio of Ki67-positive cells (red ind,e) in cultured GFP+ cells. Scale bar, 50 μm. (g–j) The presence ofCdc25andCcndsiRNAs leads to a reduction in MyoD protein (labelled with Alexa594 ing,h, arrowheads in red) and an increase in Pax7 expression (labelled with Alexa647, converted into green ing,h, arrowheads in green). Nuclei were stained with 4′,6-diamidino-2-phenylindole (DAPI) (blue). Scale bar, 20 μm. All error bars indicate ±s.e.m. (n=3).Pvalues are determined byt-test from a two-tailed distribution. *P<0.05; **P<0.01. Figure 4: miR-195/497 target Cdc25 and Ccnd messenger RNAs to induce the quiescence of MuSCs. ( a ) Effects of miR-195/497 administration on expression of genes for myogenic and cell cycle regulators in GFP+RFP+ cells isolated from diaphragms of 2-week-old mice. ( b ) Relative luciferase activity in 293T cells transfected with constructs of luciferase cDNA ligated to the 3′UTR or mutated 3′UTR (mut in Cdc25a/b , mut1~3 in Ccnd2 ) of Cdc25a , Cdc25b and Ccnd2 messenger RNAs, with or without pre-miR-497/195. ( c – f ) Introduction of mixed siRNAs against Cdc25 and Ccnd causes cell cycle exit in juvenile GFP+(RFP+) MuSCs. ( c ) Relative transcription levels of cell cycle regulators in cultured GFP+RFP+ cells of 2-week-old mice treated with or without the mixture of Cdc25 and Ccnd siRNAs are shown, indicating effective suppression of cell cycle progression with these siRNAs. ( d – f ) Effects of siRNAs against Cdc25 and Ccnd transcripts on the ratio of Ki67-positive cells (red in d , e ) in cultured GFP+ cells. Scale bar, 50 μm. ( g – j ) The presence of Cdc25 and Ccnd siRNAs leads to a reduction in MyoD protein (labelled with Alexa594 in g , h , arrowheads in red) and an increase in Pax7 expression (labelled with Alexa647, converted into green in g , h , arrowheads in green). Nuclei were stained with 4′,6-diamidino-2-phenylindole (DAPI) (blue). Scale bar, 20 μm. All error bars indicate ±s.e.m. ( n =3). P values are determined by t -test from a two-tailed distribution. * P <0.05; ** P <0.01. Full size image We next examined whether the knockdown of Cdc25a/b and Ccnd2 messenger RNAs with small interfering RNAs (siRNAs) induced quiescence of juvenile MuSCs in a manner similar to overexpression of miR-195/497 ( Supplementary Fig. 9 ). The treatment with triple siRNAs against Cdc25a/b and Ccnd2 prevented cell cycle progression of juvenile MuSCs. Knockdown of Cdc25a/b and Ccnd2 caused the simultaneous downregulation of Ccnd1 and upregulation of Cdkn2a and Cdkn1a , indicating an overall transcriptional alteration of cell cycle genes with the state of cell cyclic arrest ( Fig. 4d–f ). Moreover Cdc25a/b and Ccnd2 triple siRNA treatment increased the ratio of the Pax7+MyoD− cell population, similar to overexpression of miR-195/497 ( Fig. 4g–j ). These data indicate that Cdc25 and Ccnd2 messenger RNAs are pivotal targets of miR-195/497 in the induction of quiescence in developing MuSCs. Transplanted MuSCs with miR-195/497 enhance myogenesis Quiescent adult MuSCs are highly potent for skeletal muscle regeneration and form muscle fibres when they are transplanted into damaged muscle [26] . However, it is difficult to maintain their stemness and they lose regenerative potential when they are cultured ex vivo [16] . When adult GFP+RFP+ MuSCs isolated from diaphragms of 12 weeks old mice were cultured ex vivo , miR-195/497 expression gradually decreased along myogenic differentiation ( Fig. 5a–d ), in keeping with the functions of these miRNAs in adult quiescent MuSCs. There was an accompanying increase in the Pax7+/MyoD− population after miR-195/497 treatment, not only in juvenile MuSCs but also in adult MuSCs ( Supplementary Fig. 10 ). Exploiting the capacity of miR-195/497 to induce quiescence of proliferating MuSCs, we examined whether cultured MuSCs that proliferate can be induced to revert to quiescence and regain their regenerative activity when they are treated with miR-195/497. Dmd −/y mice were engrafted with freshly isolated GFP+RFP+ cells to evaluate the effect of cell culture with or without miR-195/497 on MuSCs transplantation. Freshly isolated GFP+RFP+ cells effectively contributed to regenerated muscle fibres after their engraftment into Dmd −/y mice, as detected by RFP expression in muscle fibres (mean=100). When cultured for 4 days ex vivo , these cells showed significantly reduced regenerative efficiency (mean=23 muscle fibres), ( Fig. 5e,f ). In contrast, when these cultured cells were transfected with miR-195/497 before transplantation, they showed more efficient regenerative myogenesis (mean=67 muscle fibres) ( Fig. 5f–h ). To compare the capacity of adult GFP+RFP+ cells, with or without miR-195/497 treatment, to renew the satellite cell compartment, we analysed numbers of GFP+ (and RFP+) cells underneath the basal lamina of skeletal muscle fibres (arrowheads in Fig. 5j ). Adult GFP+RFP+ cells transfected with miR-195/497, but not control oligonucleotides, occupied a satellite cell positions on regenerated fibres, thus indicating renewal of the satellite cell compartment (mean=0.21 GFP+ cells/RFP+ muscle fibre, Fig. 5i–k ). Conversely, the attenuation of miR-195 and miR-497 in GFP+RFP+ cells isolated from adult mice, after 24 h in culture, resulted in the elevation of transcript levels for Myogenin, MyHC, Cdc25a, Cdc25b1/2 and Ccnd2 , whereas Pax7 transcripts declined ( Fig. 6a ). We evaluated the regenerative potential of cultured MuSCs, with attenuated miR-195/497 after anti-miRNA oligo inhibitor treatment, by engraftment into Dmd −/ y mice. After 24 h culture, GFP+RFP+ cells contributed to regenerated muscle fibres after their engraftment into Dmd −/y mice, as detected by RFP expression in skeletal muscle fibres (mean=65). When cultured with miR-195/497 inhibitors, these cells showed reduced regenerative efficiency (mean=21 muscle fibres), ( Fig. 6b–f ). We conclude that miR-195 and miR-497 play an important role in maintaining the regenerative potential of MuSCs, through their effects on the cell cycle that promote a quiescent and undifferentiated state. 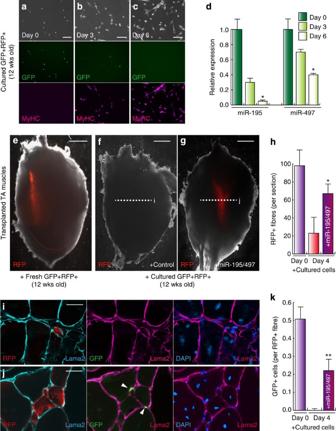Figure 5: miR-195/497 treated MuSCs have enhanced regenerative capacity. (a–c) As cultured adult GFP+RFP+ cells isolated from diaphragms of 12-week-old mice proliferate (b) and differentiate (c), GFP is shown in green and MyHC expression in pink. Scale bar, 50 μm. (d) Relative expression of miR-195/497 in cultured adult GFP+RFP+ MuSCs shown ina–c. (e–g) MyoD-primed RFP expression in TA muscles ofDmd−/ymale mice transplanted with freshly isolated (e), or cultured adult GFP+RFP+ cells without (f) or with (g) miR-195/497 for 4 days, viewed by fluorescence microscopy. Scale bar, 2.0 mm. (h) Quantification of RFP-positive fibres in TA muscles engrafted with freshly isolated (+cultured cells day 0), and cultured MuSCs with or without miR-195/497 (+cultured cells day 4). (i,j) Immunostaining for laminin (Lama2 labelled with Alexa647, pink converted into light blue) and GFP in TA muscles ofDmd−/ymice injected with cultured MuSCs treated with (j) or without (i) miR-195/497 2 weeks after intramuscular engraftment. Nuclei were stained with 4',6-diamidino-2-phenylindole (DAPI) (blue). Scale bar, 20 μm. (k) Quantification of GFP-positive cells on RFP-positive fibres with freshly isolated (day 0), and cultured MuSCs with or without miR-195/497 (day 4). All error bars indicate ±s.e.m. (n=4).Pvalues are determined byt-test from a two-tailed distribution. *P<0.05; **P<0.01. Figure 5: miR-195/497 treated MuSCs have enhanced regenerative capacity. ( a – c ) As cultured adult GFP+RFP+ cells isolated from diaphragms of 12-week-old mice proliferate ( b ) and differentiate ( c ), GFP is shown in green and MyHC expression in pink. Scale bar, 50 μm. ( d ) Relative expression of miR-195/497 in cultured adult GFP+RFP+ MuSCs shown in a – c . ( e – g ) MyoD-primed RFP expression in TA muscles of Dmd −/y male mice transplanted with freshly isolated ( e ), or cultured adult GFP+RFP+ cells without ( f ) or with ( g ) miR-195/497 for 4 days, viewed by fluorescence microscopy. Scale bar, 2.0 mm. ( h ) Quantification of RFP-positive fibres in TA muscles engrafted with freshly isolated (+cultured cells day 0), and cultured MuSCs with or without miR-195/497 (+cultured cells day 4). ( i , j ) Immunostaining for laminin (Lama2 labelled with Alexa647, pink converted into light blue) and GFP in TA muscles of Dmd −/y mice injected with cultured MuSCs treated with ( j ) or without ( i ) miR-195/497 2 weeks after intramuscular engraftment. Nuclei were stained with 4',6-diamidino-2-phenylindole (DAPI) (blue). Scale bar, 20 μm. ( k ) Quantification of GFP-positive cells on RFP-positive fibres with freshly isolated (day 0), and cultured MuSCs with or without miR-195/497 (day 4). All error bars indicate ±s.e.m. ( n =4). P values are determined by t -test from a two-tailed distribution. * P <0.05; ** P <0.01. 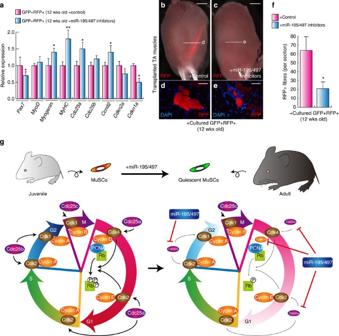Figure 6: miR-195/497 are essential for the stemness of MuSCs. (a) miR-195/497 inhibitors, added to MuSCs for 24 h, affect myogenic and cell cycle gene expression in cultured adult GFP+RFP+ cells of 12-week-old mice, as shown by qPCR analysis with the control in each case taken as 1. (b–e) MyoD-primed RFP expression (red) in TA muscles ofDmd−/ymale mice transplanted with cultured adult GFP+RFP+ cells without (b,d) or with (c,e) miR-195/497 inhibitors for 24 h, observed 2 weeks after intramuscular engraftment. Nuclei were stained with 4′,6-diamidino-2-phenylindole (DAPI) (blue). Scale bar, 2.0 mm (b,c) and 20 μm (d,e). (f) Quantification of RFP-positive fibres in engrafted TA muscles with cultured MuSCs with or without miR-195/497 inhibitors. (g) A schematic model for the regulation of skeletal MuSCs by miR-195/497. miR-195 and miR-497, members of the miR-15 family are gradually activated in MuSCs during development. These miRNAs repress the messenger RNAs for the cell cycle genes,Cdc25andCcnd, which attenuate proliferation of MuSCs by inhibiting cell cycle progression at the G1/S and G2/M phase transitions (quiescent MuSCs). All error bars indicate ±s.e.m. (n=3).Pvalues are determined byt-test from a two-tailed distribution. *P<0.05; **P<0.01. Full size image Figure 6: miR-195/497 are essential for the stemness of MuSCs. ( a ) miR-195/497 inhibitors, added to MuSCs for 24 h, affect myogenic and cell cycle gene expression in cultured adult GFP+RFP+ cells of 12-week-old mice, as shown by qPCR analysis with the control in each case taken as 1. ( b – e ) MyoD-primed RFP expression (red) in TA muscles of Dmd −/y male mice transplanted with cultured adult GFP+RFP+ cells without ( b , d ) or with ( c , e ) miR-195/497 inhibitors for 24 h, observed 2 weeks after intramuscular engraftment. Nuclei were stained with 4′,6-diamidino-2-phenylindole (DAPI) (blue). Scale bar, 2.0 mm ( b , c ) and 20 μm ( d , e ). ( f ) Quantification of RFP-positive fibres in engrafted TA muscles with cultured MuSCs with or without miR-195/497 inhibitors. ( g ) A schematic model for the regulation of skeletal MuSCs by miR-195/497. miR-195 and miR-497, members of the miR-15 family are gradually activated in MuSCs during development. These miRNAs repress the messenger RNAs for the cell cycle genes, Cdc25 and Ccnd , which attenuate proliferation of MuSCs by inhibiting cell cycle progression at the G1/S and G2/M phase transitions (quiescent MuSCs). All error bars indicate ±s.e.m. ( n =3). P values are determined by t -test from a two-tailed distribution. * P <0.05; ** P <0.01. Full size image We identified miR-195/497 as positive regulators of cell cycle quiescence in MuSCs by screening for miRNAs that are increased in these cells in adult versus developing skeletal muscle. These miRNAs induced the cell cycle arrest of proliferating juvenile MuSCs by targeting Cdc25 and Ccnd messenger RNAs. Moreover, treatment of adult MuSCs with miR-195/497 inhibitors caused activation of mRNAs for Cdc25 and Ccnd and decreased expression of Pax7 while overexpression of miR-195/497 in MuSCs increased Pax7+ cells. On the other hand, in silico analyses show no evidence for direct targeting of Pax7 or MyoD transcripts by miR-195/497, suggesting that these transcription factors are not direct targets of miR-195/497. Taken the effects of the attenuation of Cdc25 and Ccnd on an increased ratio of Pax7+/MyoD− cell populations in MuSCs ( Fig. 4g–j ) into consideration, our data support an idea that miR-195/497 mediate quiescence of MuSCs through targeting genes for cell cycle progression, which results in an increase in Pax7+ MuSC population ( Fig. 6g ). The cell cycle arrest induced by expression of miR-195/497 or by knockdown of Cdc25/Ccnd transcripts not only elicited the upregulation of Pax7 and the downregulation of MyoD protein, characteristics of quiescent adult MuSCs, but also enhanced the regenerative potential of cultured adult MuSCs and their integration into the stem cell niche after their engraftment. Conversely, prolonged periods of cell culture and miR-195/497 inhibitors decreased the regenerative myogenesis of adult MuSCs ( Figs 5f and 6b ). These results suggest that a close link between cell cycle withdrawal and quiescence induced by miR-195/497 and the regenerative potential of MuSCs. Our miRNA screening detected upregulation of not only miR-195/497 but also miR-29, miR-126, and miR-489 in adult MuSCs. miR-489 was described previously by Cheung et al. They compared miRNAs expressed in quiescent and activated adult MuSCs and found that miR-489 is essential for the maintenance of stem cell quiescence through the suppression of Dek posttranscriptionally. Although Dek has been characterized as a non-histone nuclear protein and therefore considered as a transcriptional modulator of cell division of MuSCs, recent studies suggest that it also functions as a secreted molecule [27] . It remains to be seen whether miR-195/497 cooperate with miR-489 to arrest the cell cycle of MuSCs. In contrast, a number of miRNAs, including miR-1, miR-206 and miR-27, participate in skeletal muscle differentiation. These miRNAs repress the expression of Pax3 and Pax7 proteins, and promote the proliferation and differentiation of MuSCs [21] , [28] , [29] . Thus, miR-195/497 and miR-1/206/27 are implicated in the quiescent and activated states of MuSCs, respectively. Porrello et al. [30] showed that the miR-15 family, expressed in differentiated postnatal cardiomyocytes, induces cell cycle arrest through targeting the messenger RNA of the cell cycle gene Chek1 (checkpoint kinase 1) and that high levels of miR-195 contribute to loss of the regenerative capacity of hearts after birth [31] . In this case, the induction of cell cycle arrest caused by the activation of miR-195 appears to result in the progression of terminal differentiation of cardiomyocytes. Thus, whether cell cycle arrest caused by the miR-15 family induces the quiescence of stem cells or promotes terminal differentiation may be dependent on the cellular context. We also note that Cdc25 and Ccnd messenger RNAs that are targets of miR-195/497 likely also play a role in cell cycle withdrawal before terminal myogenic differentiation. The downregulation of Cdc25 in differentiating C2C12 myoblasts in the presence of miR-322/424 and miR-503 promotes cell cycle arrest necessary for terminal differentiation, while the downregulation of Ccnd2 in neonatal myoblasts enhances muscle cell fusion [32] , [33] . It remains to be seen whether miR-195/497 are also involved in cell cycle arrest during the terminal differentiation of myoblasts, and whether MuSCs require similar miRNA regulation of Cdc25/Ccnd mRNAs to form skeletal muscle fibres. In all experiments we used Pax3GFP; MyoD-primed RFP mice to identify skeletal MuSCs. The percentage of GFP+RFP+ cells increases during prenatal stages and immediately after birth ( Fig. 1a ), so that very few cells of the GFP+RFP− population are present in adult skeletal muscle where they represent less than 3% of total GFP+ cells (right panel in Fig. 1a ). Further investigation would be required to see whether this small fraction of cells has distinct properties, as discussed for Pax7+Myf5− satellite cells [13] , and other posttranscriptional regulatory mechanisms that miR-195/497 target Cdc25 and Ccnd . Finally, we raise the question of possible therapeutic applications of miR-195/497. Novel therapies based on stem cell transplantation include those for genetic disorders, such as DMD, and will require the expansion of stem cells ex vivo . Cultured MuSCs progress towards myogenesis, with accumulation of MyoD protein, and have reduced regenerative potential [14] , [16] . Consistently, early clinical trials involving the transplantation of ex vivo expanded myogenic cells have failed to improve strength in patients with DMD [34] . Our data suggest that the quiescent state of MuSCs raises the regenerative myogenic potential although reasons for it need to be elucidated. In addition to MuSCs, it is likely that there will be demand for MuSC induction from pluripotent stem cells, with attempts to maintain the stemness of MuSC with growth factors, chemicals or substrate elasticity [35] , [36] , [37] . In this context, it is noteworthy that transient introduction of miR-195/497 into cultured MuSCs sustained their stemness and enhanced their regenerative potential on transplantation into DMD model mice. Thus, further investigation of the characteristics of MuSCs, including molecular mechanisms underlying their establishment and maintenance in adult muscle, has the potential to open up new perspectives for stem cell therapies of skeletal muscle disorders. Mouse lines Pax3 GFP/+ , Pax7 CreER/+ , MyoD-Cre-IRES-nlacZ ( MyoD-Cre ), Rosa26 CAG-LSL-RFP/+ (Jackson Laboratory; stock number 007914, LSL ; loxP-stop-loxP), Dcr f/+ ( Dicer floxed/+ ) and Dmd −/y mouse lines were used [2] , [15] , [38] , [39] , [40] . 4-hydroxytamoxifen (Sigma) was administrated to 12 weeks old male mice at 1.0 mg per 40 g body weight intraperitoneally for five straight days. All animal experiments were carried out according to the Regulations of Animal Experimentation of Kyoto University. Cell sorting and cell culture For live cell sorting and culture, skeletal muscle tissue was treated with 0.1% collagenase (Sigma) and 0.1% trypsin (Gibco) in DMEM/F12 supplemented with GlutaMax (Gibco) at 37 °C for 2 h. Dissociated cells were resuspended with 1% bovine serum albumin in Hank’s Balanced Salt Solution buffer (Gibco) and filtrated with cell strainer (BD). Cell suspensions were stained with 1 μg ml −1 propidium iodide to exclude dead cells and calculate cell cycle phases. For transfection with each 50 nM of mir Vana miRNA mimics, mir Vana miRNA inhibitors (Ambion) or MISSION siRNAs (Sigma) listed in Supplementary Table 2 , isolated cells were incubated with Lipofectamine RNAiMAX (Invitrogen) according to manufacture protocols of the reverse transfection for 24 h, followed by changing of the culture media. The Luciferase assay was performed with pmirGLO Dual-Luciferase miRNA Target Expression Vector (Promega) transfected 293T cells by using the Dual-Luciferase Reporter Assay System (Promega) with a GloMax 20/20 luminometer (Promega). miRNA microarray and RT–qPCR analyses Total RNAs from sorted or cultured cells were extracted using miRNeasy Micro Kit (Qiagen). For miRNA microarray analyses, biotin-labelled RNA was prepared using FlashTag HSR RNA labelling kit (Genisphere), and hybridization to GeneChip miRNA2.0 Array (Affymetrix) was performed according to Affymetrix protocols. Hybridized arrays were scanned using an Affymetrix GeneChip Scanner. The data analyses were performed using Expression Console (Affymetrix) and GeneSpring GX software (Agilent Technologies). For quantitative PCR analyses, synthesized cDNA was prepared using SuperScript III kit (Invitrogen) with random hexamers from mRNAs or miScript RT kit (Qiagen) from mature miRNAs. All RT–qPCR reactions were carried out in triplicate using Power SYBR Green PCR Master Mix (Applied Biosystems), and normalized to mRNA expression level of ribosomal protein L13A (Rpl13a) or non-coding RNA expression level of U6 small nuclear RNA as a control. Primer sequences (5′ to 3′) are listed in Supplementary Table 1 . Immunofluorescence Cells and skeletal muscle tissues were fixed with 1% paraformaldehyde, 0.1% Triton X-100 in PBS for 60 min at 4 °C, before embedding in Frozen Section Compound (Leica Microsystems) for cryosections. Fixed samples were incubated with anti-GFP (Molecular Probes; diluted 1/500), anti-ß-galactosidase (Sigma; diluted 1/200), anti-Pax3 (DSHB; diluted 1/100), anti-Pax7 (DSHB; diluted 1/100), anti-MyoD (DAKO; diluted 1/100), anti-MyHC (R&D; diluted 1/200), anti-Laminin (Enzo Life Sciences; diluted 1/500), anti-active Caspase3 (BD Pharmingen; diluted 1/200), anti-pHH3 (Cell Signaling Technology; diluted 1/200) and anti-Ki67 (DAKO; diluted 1/200) antibodies in 5% of BlockingOne (Nacalai) for overnight at 4 °C. EdU incorporations were assayed according to manufacture protocol (Molecular Probes; Click-iT EdU Imaging Kit). After three washes with 0.05% of Tween20 in PBS, cells were incubated with Alexa488, Alexa594 or Alexa647-conjugated secondary antibodies (Molecular Probes; diluted 1/500). Cells were washed and mounted in ProLong Gold antifade reagent with DAPI (Molecular Probes). Images were collected and processed to change original fluorescent colours when appropriate on the software of BioZero (Keyence) and ApoTome (Carl Zeiss). For quantitation of cultured cells, numbers of dishes were analysed from triplicate experiments. Grafting of MuSCs into dystrophin-deficient muscle tissues Twelve weeks or older Dmd −/y host male mice were used for engraftment of freshly isolated or cultured MuSCs (1.0 × 10 4 cells per 20 μl of PBS) into tibialis anterior (TA) muscle fibres. Mice were anesthetized with diethyl ether before engraftment. TA muscle was removed 2 weeks after transplantation, fixed and stained as above. For quantification, serial transverse sections were cut across the entire TA muscle generating about 20 slides per muscle where each slide contains about 20 serial sections. Five different slides were immunostained, covering regions where most engrafted cells were present. At least four transplanted mice were analysed per each experiment. Statistics We report the statistical data, including results of at least three biological replicates. Statistical analyses were performed with StatPlus software (AnalystSoft) to determine significant differences from a two-tailed distribution using paired or unpaired Student’s t -test. P values indicated on each figure as <0.05 (*), <0.01 (**) and <0.001 (***). All error bars are indicated as means±s.e.m. Accession codes : The microarray data have been deposited in Gene Expression Omnibus under accession number GSE48412 . How to cite this article : Sato, T. et al. miR-195/497 induce postnatal quiescence of skeletal muscle stem cells. Nat. Commun. 5:4597 doi: 10.1038/ncomms5597 (2014).